A crucial role for bone morphogenetic protein-Smad1 signalling in the DNA damage response DNA damage and the elicited cellular response underlie the etiology of tumorigenesis and ageing. Yet, how this response integrates inputs from cells' environmental cues remains underexplored. Here we report that the BMP-Smad1 pathway, which is essential for embryonic development and tissue homeostasis, has an important role in the DNA damage response and oncogenesis. On genotoxic stress, Atm phosphorylates BMPs-activated Smad1 in the nucleus on S239, which disrupts Smad1 interaction with protein phosphatase PPM1A, leading to enhanced activation and upregulation of Smad1. Smad1 then interacts with p53 and inhibits Mdm2-mediated p53 ubiquitination and degradation to regulate cell proliferation and survival. Enhanced Smad1 S239 phosphorylation, and Smad1 mutations causing S239 substitution were detected in oesophageal and gastric cancer samples, respectively. These findings suggest that BMP-Smad1 signalling participates in the DNA damage response via the Atm-p53 pathway, thus providing a molecular mechanism whereby BMP-Smad1 loss-of-function leads to tumorigenesis, for example, juvenile polyposis and Cowden syndromes. The genome is under constant attack by endogenous factors such as mitochondria-generated reactive oxygen species and DNA replicative stress, and exogenous factors such as ionizing radiation (IR) and chemotherapeutic drugs. DNA damage underlies the development of both cancer and ageing. Mammalian cells have evolved a complex network to detect and cope with DNA damage. At the centre of the DNA damage response (DDR) lie the PI3-Kinase-like kinases including Atm and Atr, which activate p53 and other substrates to constrain cell propagation [1] , [2] , [3] . Recent studies indicate that the DDR is also activated during precancerous to cancerous transition [4] , [5] , [6] , acting as a barrier of tumorigenesis. Eventually, mutations arise in DDR genes, leading to cell transformation, for example, p53 is inactivated in more than 50% of human cancers [7] . An understanding of the full breadth of cell response to DNA damage, including the contribution of cells' environmental signals, helps to identify new cancer therapy targets. Bone morphogenetic proteins (BMPs) are essential regulators of early development and homeostasis of various adult tissues [8] , [9] , [10] , [11] , [12] , [13] . The binding of BMPs to the BMP receptor I (BMPRI) and II complex leads to the activation of BMPRI, which phosphorylates Smad1/5/8 at the Carboxy-terminal SXS motif (activation). SXS phosphorylation is essential for Smad1 nuclear entry, where they bind to the Smad-binding element of target genes to regulate transcription [13] , [14] . On the completion of transcriptional regulation, Smad1 activation is terminated by multiple mechanisms, including removal of SXS phosphorylation by phosphatases, for example, PPM1A, in the nucleus [15] , which promotes nuclear export of Smads [14] , [16] . Besides the SXS motif, the linker region located between the MH1 (Mad homology 1, the DNA-binding domain) and MH2 of Smad proteins can be phosphorylated by MAPKs, CDK, or GSK3, and phosphorylation was shown to negatively regulate Smad activity [17] , [18] , [19] . Human and mouse genetic studies reveal a tumour suppressor function for the BMP-Smad pathway [20] . Mutations in BMPRIA have been linked to the development of juvenile polyposis syndrome and Cowden syndrome in human, and deactivation of BMP-Smad pathway has been found in the majority of sporadic colorectal cancers [21] , [22] , [23] , [24] . Conventional deletion of BMPRIA, Smad1 or Smad5 results in embryonic lethality in mice [25] , while conditional deletion of BMPRIA in ventral limb ectoderm and intestinal epithelial cells resulted in skin tumours and polyposis, respectively, and conditional deletion of both Smad1 and Smad5 in the somatic cells of gonads leads to metastatic tumour development [26] , [27] . Yet, little is known about how BMP-Smad1 pathway suppresses tumorigenesis. Tumour suppression can be achieved by suppressing oncogenic pathways, maintaining genome integrity, inhibiting cell division, promoting apoptosis, or promoting differentiation. Here we report that the BMP-Smad pathway is a part of the DDR and that Atm-mediated Smad1 S239 phosphorylation has critical roles in p53 induction, DDR, and tumorigenesis, thus providing a mechanistic explanation pertaining to the tumour suppression activity of BMP-Smad signalling and expanding our knowledge of the DDR. DNA damage leads to Atm-dependent Smad1 activation Our previous mouse studies revealed a role for Atm, c-Abl and p53, three players in DDR, in bone homeostasis and osteoblastogenesis, by regulating the expression of osteoblast-specific transcription factor Osterix [28] , [29] , [30] . Osterix is a target gene of the BMP-Smad pathway and this link prompted us to question whether the BMP-Smad pathway is involved in the cell response to DNA damage. Under normal culture conditions, mouse embryonic fibroblasts (MEFs) and other examined cell types showed basal levels of Smad1/5/8 activation and expression of BMP target gene Id1, due to autocrine or serum-containing BMPs, which could be inhibited by BMP antagonists noggin and chordin ( Supplementary Fig. S1a ). Treatment with genotoxic drugs, such as Doxorubicin (Dox), enhanced the activation of Smad1/5/8, but not the TGFβ-responsive Smad2/3 in MEFs, and this was accompanied by an upregulation of total Smad1, but not Smad5 or Smad8 ( Fig. 1a ). Moreover, Smad1 activation and upregulation were also observed in Ras V12 /E1A-transformed MEFs, and mouse ES cells in response to Dox, hydroxyurea or IR ( Supplementary Figs S1b–d ). Like BMP2 treatment, DNA damage also induced an increase in the levels of nuclear Smad1, as judged by immunohistochemistry assays ( Fig. 1b ). Like BMP2, Dox treatment activated only a portion of Smad1. Moreover, microarray analysis revealed that about 50% of the BMP2-activated genes were also activated by Dox treatment in primary MEFs, Ras V12 /E1A-transformed MEFs, and mouse ES cells ( Fig. 1c ), supporting the conclusion that genotoxic stress could activate BMP-Smad1 signalling. 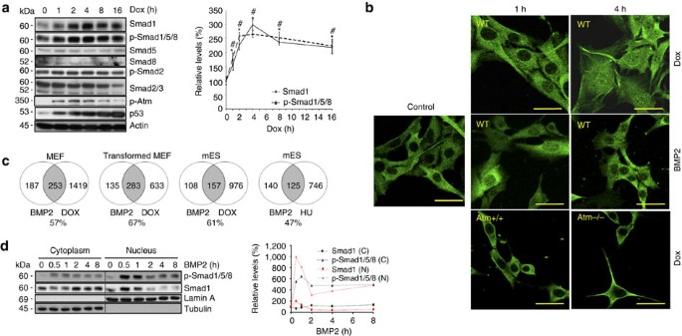Figure 1: Genotoxic stress led to enhanced Smad1 SXS phosphorylation and upregulation. (a) Dox induced Smad1/5/8 activation and upregulation of Smad1, but not of Smad5, 8, 2 and 3, in MEFs. Primary MEFs were treated with 1 μM Dox for different periods of time. Activation of Smads and their protein levels were analysed by western blot. Right panel: quantitation of p-Smad1/5/8 and Smad1 that was normalized to actin. The levels of Smad1 or p-Smad1 at time 0 were set at 100%. All data were presented as means±s.e.m. (n=3) and were statistically assessed using Student'st-test. *P<0.05 when Smad1 was compared with that of time 0. #P&<0.05 when p-Smad1/5/8 was compared with that of time 0. Activation of Atm and induction of p53 were used as indication of DNA damage. (b) Immuno-staining shows that DNA damage induced Smad1 elevation in the nucleus, in Atm-dependent manner. MEFs (WT andAtm−/−) with stable expression of Smad1 by retrovirus were treated with Dox or 50 ng ml−1BMP2 for different periods of time. The cells were immunostained with antibodies against Smad1 and then FITC-conjugated secondary antibodies. Scale bar, 20 μm. (c) Microarray analysis of gene expression profiles of three cell types. Primary MEFs were treated with BMP2 (100 ng ml−1) or Dox (1.0 μM) for 16 h. Transformed MEFs were treated with BMP2 (100 ng ml−1) or Dox (0.3 μM) for 12 h. Mouse ES cells were treated with BMP2 (100 ng ml−1), Dox (0.2 μM) or HU (5 mM) for 18 h. Genes whose induction was >2.0 fold were analysed. Transformed MEFs were generated by expression of RasV12/E1A in primary MEFs with retroviruses. Percentage of genes induced by both Dox and BMP2 to total BMP2-induced genes was presented. (d) BMP2 transiently activates Smad1/5/8 in both cytoplasm and nucleus. MEFs were treated with 50 ng ml−1BMP2 for various time periods. Cells were then collected and separated into cytoplasmic and nuclear fractions. Smad1/5/8 phosphorylation and Smad1 were analysed by WB. Right panel: quantification data. Figure 1: Genotoxic stress led to enhanced Smad1 SXS phosphorylation and upregulation. ( a ) Dox induced Smad1/5/8 activation and upregulation of Smad1, but not of Smad5, 8, 2 and 3, in MEFs. Primary MEFs were treated with 1 μM Dox for different periods of time. Activation of Smads and their protein levels were analysed by western blot. Right panel: quantitation of p-Smad1/5/8 and Smad1 that was normalized to actin. The levels of Smad1 or p-Smad1 at time 0 were set at 100%. All data were presented as means±s.e.m. ( n =3) and were statistically assessed using Student's t -test. * P <0.05 when Smad1 was compared with that of time 0. # P &<0.05 when p-Smad1/5/8 was compared with that of time 0. Activation of Atm and induction of p53 were used as indication of DNA damage. ( b ) Immuno-staining shows that DNA damage induced Smad1 elevation in the nucleus, in Atm-dependent manner. MEFs (WT and Atm −/− ) with stable expression of Smad1 by retrovirus were treated with Dox or 50 ng ml −1 BMP2 for different periods of time. The cells were immunostained with antibodies against Smad1 and then FITC-conjugated secondary antibodies. Scale bar, 20 μm. ( c ) Microarray analysis of gene expression profiles of three cell types. Primary MEFs were treated with BMP2 (100 ng ml −1 ) or Dox (1.0 μM) for 16 h. Transformed MEFs were treated with BMP2 (100 ng ml −1 ) or Dox (0.3 μM) for 12 h. Mouse ES cells were treated with BMP2 (100 ng ml −1 ), Dox (0.2 μM) or HU (5 mM) for 18 h. Genes whose induction was >2.0 fold were analysed. Transformed MEFs were generated by expression of Ras V12 /E1A in primary MEFs with retroviruses. Percentage of genes induced by both Dox and BMP2 to total BMP2-induced genes was presented. ( d ) BMP2 transiently activates Smad1/5/8 in both cytoplasm and nucleus. MEFs were treated with 50 ng ml −1 BMP2 for various time periods. Cells were then collected and separated into cytoplasmic and nuclear fractions. Smad1/5/8 phosphorylation and Smad1 were analysed by WB. Right panel: quantification data. Full size image BMPs are synthesized and secreted by many cell types including ES cells, and exist in the niche of some somatic stem cell types as well as the bloodstream (reviewed in ref. 8 ). BMPs-activated Smad1 is also accompanied by a modest upregulation of Smad1 in MEFs ( Fig. 1d ). However, BMP2 alone could not induce DDR, as it exhibited no discernible effects on p53 or its target genes ( Mdm2, p21 and Bax ) in MEFs ( Fig. 2a,b ). Comparison of Smad1 activation kinetics revealed that genotoxic stress induced sustained Smad1 nuclear localization and upregulation ( Fig. 2c ), whereas BMP2 treatment led to a transient increase of Smad1 in the nucleus, followed by a rapid decrease (lower-than-basal level) ( Fig. 1d ), as previously reported (reviewed in ref. 8 ). Moreover, Dox-induced Smad1 activation and upregulation mainly occurred in the nucleus, with the change in cytoplasm being rather modest ( Fig. 2c ). 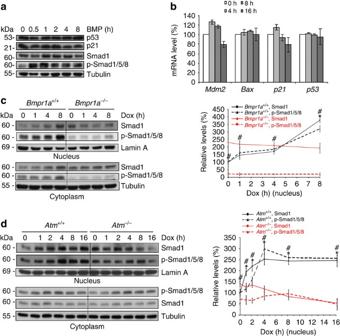Figure 2: BMPs and Atm were required for full Smad1 activation/upregulation under genotoxic stress. (a,b). BMP2 does not activate p53. Primary MEFs were challenged with 50 ng ml−1of BMP2 for various periods of time. p53 and p21 were assessed by western blot analysis (a), and mRNA levels of p53 and its target genes Mdm2, p21 and Bax were determined by real-time PCR (b). (c).Bmpr1a−/−ES cells showed diminished Smad1 activation and upregulation under genotoxic stress, mainly in the nucleus.Bmpr1a−/−and control normal ES cells were treated with 0.2 μM Dox and fractionated into cytoplasm and nuclear portions. Right panel: quantification of p-Smad1/5/8 and Smad1 that was normalized to lamin A. The levels of Smad1 or p-Smad1 at time 0 for WT cells were set at 100%. All data were presented as mean±s.e.m. (n=3) and were statistically assessed using Student'st-test. *P<0.05 when Smad1 inBmapr1a−/−was compared (less) with that of WT cells. #P<0.05 when p-Smad1/5/8 inBmapr1a−/−cells was compared with that of WT cells. (d). Activation and elevation of Smad1 mainly occurred in the nucleus in an Atm-dependent manner. WT andAtm−/−MEFs were treated with Dox for different periods of time and then fractionated into the cytoplasmic and nuclear fractions. Right panel: quantification of p-Smad1/5/8 and Smad1 that was normalized to lamin A. The levels of Smad1 or p-Smad1 at time 0 for WT cells were set at 100%. All data were presented as mean±s.e.m. (n=3) and were statistically assessed using Student'st-test. *P<0.05 when Smad1 inAtm−/−cells was compared with that inAtm+/+cells. #P<0.05 when p-Smad1 inAtm−/−cells was compared with that inAtm+/+cells. Figure 2: BMPs and Atm were required for full Smad1 activation/upregulation under genotoxic stress. ( a,b ). BMP2 does not activate p53. Primary MEFs were challenged with 50 ng ml −1 of BMP2 for various periods of time. p53 and p21 were assessed by western blot analysis ( a ), and mRNA levels of p53 and its target genes Mdm2, p21 and Bax were determined by real-time PCR ( b ). ( c ). Bmpr1a −/− ES cells showed diminished Smad1 activation and upregulation under genotoxic stress, mainly in the nucleus. Bmpr1a −/− and control normal ES cells were treated with 0.2 μM Dox and fractionated into cytoplasm and nuclear portions. Right panel: quantification of p-Smad1/5/8 and Smad1 that was normalized to lamin A. The levels of Smad1 or p-Smad1 at time 0 for WT cells were set at 100%. All data were presented as mean±s.e.m. ( n =3) and were statistically assessed using Student's t -test. * P <0.05 when Smad1 in Bmapr1a −/− was compared (less) with that of WT cells. # P <0.05 when p-Smad1/5/8 in Bmapr1a −/− cells was compared with that of WT cells. ( d ). Activation and elevation of Smad1 mainly occurred in the nucleus in an Atm-dependent manner. WT and Atm −/− MEFs were treated with Dox for different periods of time and then fractionated into the cytoplasmic and nuclear fractions. Right panel: quantification of p-Smad1/5/8 and Smad1 that was normalized to lamin A. The levels of Smad1 or p-Smad1 at time 0 for WT cells were set at 100%. All data were presented as mean±s.e.m. ( n =3) and were statistically assessed using Student's t -test. * P <0.05 when Smad1 in Atm −/− cells was compared with that in Atm +/+ cells. # P <0.05 when p-Smad1 in Atm −/− cells was compared with that in Atm +/+ cells. Full size image Importantly, the presence of BMPs in the culture medium and Smad1 SXS phosphorylation were prerequisites for enhanced Smad1 activation and upregulation by genotoxic stress, as BMPRIA deficiency or SXS deletion diminished Dox-augmented Smad1 SXS phosphorylation and led to a downregulation of Smad1 in the nucleus, but at a reduced extent in the cytoplasm ( Fig. 2c ; Supplementary Fig. S2a ). The Smad1 was higher at basal levels under these two conditions likely due to feedback regulation, yet Smad proteins are not functional without SXS phosphorylation [13] . Thus, BMP-induced Smad1 SXS phosphorylation is necessary for Dox-induced Smad1 upregulation in the nucleus, and that BMPs' presence is necessary for Dox-induced enhancement of Smad1 activation. We next tested whether Atm, whose activation is among the earliest events of DDR, is required for Smad1 activation/upregulation under genotoxic stress. It was found that Dox-induced nuclear Smad1 SXS phosphorylation was inhibited and the nuclear Smad1 protein levels were reduced in Atm −/− MEFs ( Fig. 2d ). The effects of Atm deficiency on cytoplasmic Smad1 were rather modest ( Fig. 2d ). Inhibition of PI3-Kinase-like kinases with caffeine also diminished Dox-induced Smad1 activation and upregulation ( Supplementary Fig. S2b ). These results suggest that Atm has an important role in Smad1 activation/upregulation, especially in the nucleus, under genotoxic stress. Atm phosphorylates Smad1 on S239 in the nucleus Smad1 SXS phosphorylation is positively regulated by BMPs and BMPRs and negatively regulated by protein phosphatases. Microarray analysis revealed that Dox treatment did not alter the messenger RNA levels of BMP ligands and receptors. Real-time PCR analysis confirmed that expression of the major activators of Smad1, including BMP2 , 4 , 6 and 7 and BMPRIA and II , was not significantly affected by Dox ( Supplementary Fig. S2c ). In addition, Dox, unlike BMP2, did not upregulate Smad6 and Smad7 , the I-Smads ( Supplementary Fig. S2d ). Although Atm is required for Dox-induced Smad1 activation and upregulation, Atm deficiency did not alter the expression of BMP2 , 4 , 6 , 7 and BMPRIA and II ( Supplementary Fig. S2e ). In addition, Dox treatment did not affect the kinase activity of BMPRIA towards Smad1 ( Supplementary Fig. S2f ). These results, together with the finding that only Smad1 is upregulated in response to Dox ( Fig. 1a ), suggest that DNA damage might act on Smad1, probably SXS dephosphorylation, rather than the upstream BMP ligands and receptors. Atm phosphorylates p53, Chk2 and other substrates on S/TQ motifs, which can be recognized by anti-p-S/TQ antibodies [31] , [32] . Co-expression experiments indicated that Atm was able to phosphorylate Smad1, which contains predicted S/TQ motifs, including S239 in the linker region ( Supplementary Fig. S3a ), although Smad1 and Atm did not form a stable complex ( Fig. 3a ). Atm did not phosphorylate BMPRIA, BMPRIB or BMPRII. Site-directed mutagenesis of S 239 Q to AQ, a site located in the linker region of Smad1 and Smad5 but not in Smad8, Smad2 or Smad3, abolished this phosphorylation, whereas substitution of T 452 Q to AQ, a site conserved among Smad1/2/3/5/8 at the MH2 domain, had no such effect ( Fig. 3a ; Supplementary Fig. S3a ). We generated polyclonal antibodies against S239-phosphorylated Smad1 and confirmed its specificity with wild type (WT) and S239A mutant Smad1 expressed in the presence or absence of Atm ( Supplementary Fig. S3b ). Using this antibody, we showed Dox treatment led to an increase in S239 phosphorylation of endogenous Smad1 ( Fig. 3b ), and Atm −/− MEFs showed little Smad1 S239 phosphorylation in response to Dox ( Fig. 3c ). In vitro kinase assays confirmed that Atm, but not the kinase-dead Atm, could phosphorylate bacteria-expressed Smad1 ( Fig. 3d ), suggesting that Smad1 is an Atm substrate. Similar to Dox-induced Smad1 activation/upregulation, Dox-induced S239 phosphorylation mainly occurred in the nucleus ( Supplementary Fig. S3c ) and required Smad1 SXS phosphorylation, as noggin and chordin treatment or SXS deletion diminished Smad1 S239 phosphorylation ( Fig. 3a ; Supplementary Fig. S3d ). Atm was also required, as caffeine pretreatment or Atm deficiency diminished S239 phosphorylation ( Fig. 3c ; Supplementary Fig. S3d ). By contrast, Atm did not seem to phosphorylate the highly homologous Smad5 on this SQ motif ( Supplementary Fig. S3e ), probably due to the presence of a polar amino-acid Asn in front of SQ [33] . 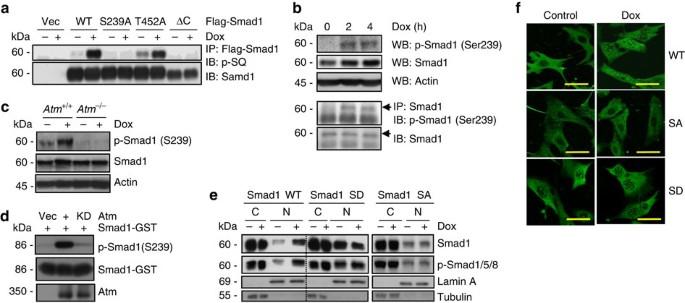Figure 3: Atm phosphorylated Smad1 at S239 and was necessary for Smad1 activation and upregulation. (a). Phosphorylation of Smad1 at S/TQ motif by Atm occurs at S239 but not T452. Flag-tagged Smad1, Smad1 S239A, Smad1 T452A, or Smad1ΔC, together with Atm, were expressed in 293T cells, which were treated with Dox for 4 h before collection. Smad1 was immunoprecipitated and their S/TQ phosphorylation was determined by western blot. (b). Dox induced SQ phosphorylation of endogenous Smad1. MEFs were treated with or without Dox. Upper panel: S239 phosphorylation of endogenous Smad1 was directly detected with western blot using the newly developed anti-phospho-S239 Smad1 antibodies. Lower panel: the immunoprecipitated endogenous Smad1 could also be recognized by the new antibodies. (c). Smad1 S239 phosphorylation was significantly inhibited inAtm−/−MEFs. WT andAtm−/−MEFs were treated with Dox for 2 h, and the S239 phosphorylation was determined by western blot. (d). Atm was able to phosphorylate bacteria-expressed Smad1in vitro. Flag-tagged Atm or kinase dead Atm was expressed in 293T cells and enriched by immunoprecipitation. GST-Smad1, which was expressed in and purified from bacteria, was used as a substrate. Smad1 S239 phosphorylation was detected by Western blot analysis using anti-p-Smad1 S239 antibodies. (e). Dox-induced Smad1 activation and nuclear elevation required S239 phosphorylation. MEFs expressing WT, S239A, or S239D Smad1 were treated with Dox and fractionated into cytoplasmic (C) and nuclear (N) fractions for western blot analysis. (f). S239A mutation diminished Dox-induced Smad1 nuclear elevation while S239D mutation promoted it. Flag-tagged Smad1 of WT, SA or SD mutant forms was expressed inSmad1−/−MEFs with retrovirus and immunostained with anti-Flag antibodies. Scale bar, 20 μm. Figure 3: Atm phosphorylated Smad1 at S239 and was necessary for Smad1 activation and upregulation. ( a ). Phosphorylation of Smad1 at S/TQ motif by Atm occurs at S239 but not T452. Flag-tagged Smad1, Smad1 S239A, Smad1 T452A, or Smad1ΔC, together with Atm, were expressed in 293T cells, which were treated with Dox for 4 h before collection. Smad1 was immunoprecipitated and their S/TQ phosphorylation was determined by western blot. ( b ). Dox induced SQ phosphorylation of endogenous Smad1. MEFs were treated with or without Dox. Upper panel: S239 phosphorylation of endogenous Smad1 was directly detected with western blot using the newly developed anti-phospho-S239 Smad1 antibodies. Lower panel: the immunoprecipitated endogenous Smad1 could also be recognized by the new antibodies. ( c ). Smad1 S239 phosphorylation was significantly inhibited in Atm −/− MEFs. WT and Atm −/− MEFs were treated with Dox for 2 h, and the S239 phosphorylation was determined by western blot. ( d ). Atm was able to phosphorylate bacteria-expressed Smad1 in vitro . Flag-tagged Atm or kinase dead Atm was expressed in 293T cells and enriched by immunoprecipitation. GST-Smad1, which was expressed in and purified from bacteria, was used as a substrate. Smad1 S239 phosphorylation was detected by Western blot analysis using anti-p-Smad1 S239 antibodies. ( e ). Dox-induced Smad1 activation and nuclear elevation required S239 phosphorylation. MEFs expressing WT, S239A, or S239D Smad1 were treated with Dox and fractionated into cytoplasmic (C) and nuclear (N) fractions for western blot analysis. ( f ). S239A mutation diminished Dox-induced Smad1 nuclear elevation while S239D mutation promoted it. Flag-tagged Smad1 of WT, SA or SD mutant forms was expressed in Smad1 −/− MEFs with retrovirus and immunostained with anti-Flag antibodies. Scale bar, 20 μm. Full size image S239 phosphorylation promotes Smad1 activation/upregula-tion We generated a Smad1 S239A mutant that is resistant to phosphorylation and a S239D mutant that mimics phosphorylation and expressed them in Smad1 −/− MEFs with retroviral vectors. Dox led to nuclear upregulation and SXS phosphorylation of WT Smad1, but much less of Smad1 S239A ( Fig. 3e,f ). On the other hand, the Smad1 S239D mutant showed enhanced activation and more nuclear localization at the basal level ( Fig. 3e,f ). Taken together, these results indicate that Atm-mediated S239 phosphorylation is required for effective Smad1 activation and upregulation by genotoxic stress, this is in contrast to Smad linker phosphorylation mediated by CDK and MAPKs, which seem to have a negative effect on Smad1 activity [18] . Further studies show that Dox-induced S239 phosphorylation might enhance Smad1 activation by delaying Smad1 SXS dephosphorylation in the nucleus. As previously described, washing out the medium-containing BMPs would allow Smad1 to be dephosphorylated on SXS [34] . We found that Dox-pretreatment inhibited this dephosphorylation process (more than threefold increase in T 1/2 ), especially in the nucleus, without affecting Smad2 ( Fig. 4a ; Supplementary Fig. S4 ). These results suggest that protein phosphatases responsible for Smad1 SXS dephosphorylation may be involved in Dox-induced Smad1 activation and upregulation. 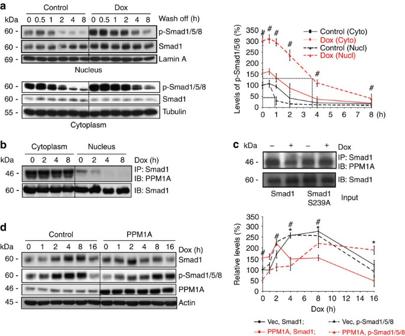Figure 4: DNA damage impeded SXS dephosphorylation by interfering with Smad1–PPM1A interaction. (a). DNA damage inhibited the dephosphorylation of nuclear Smad1/5/8. MEFs were treated with Dox for 4 h and then cultured in serum-free medium for different periods of time. The cells were collected and fractionated into cytoplasmic and nuclear fractions. Right panel: quantification of p-Smad1/5/8 that was normalized to lamin A or tubulin. The level of p-Smad1 at time 0 for untreated cells were set at 100%. All data were presented as mean±s.e.m. (n=3) and were statistically assessed using Student'st-test. #P<0.05 when the level of p-Smad1 in Dox-treated cells was compared with that in untreated cells. (b) DNA damage inhibited the interaction between PPM1A and Smad1. MEFs were treated with Dox for different periods of time, collected and fractionated into the cytoplasmic and nuclear fractions, and then Smad1 was immunoprecipitated. Co-immunoprecipitated PPM1A was detected by western blot. (c) DNA damage inhibited the interaction between PPM1A and Smad1 in a S239 dependent manner. Flag-tagged Smad1 or Smad1S239A was expressed in 293T cells, which were treated with Dox for 6 h, and nuclear fractions were immunoprecipitated with anti-Flag conjugated beads. Same amounts of purified PPM1A proteins were added to the beads carrying Smad1 and incubated overnight. The bound PPM1A was detected by western blot. (d) Overexpression of PPM1A inhibited DNA damage-induced Smad1 upregulation. MEFs were infected with retrovirus expressing PPM1A, selected for 3 days, and then treated with Dox. Smad1 and p-Smad1 were detected by western blot analysis. Right panel: quantification of p-Smad1/5/8 and Smad1 that was normalized to actin. The levels of Smad1 or p-Smad1 at time 0 for vector-infected cells were set at 100%. All data were presented as mean± s.e.m. (n=3) and were statistically assessed using Student'st-test. *P<0.05 when Smad1 in PPM1A-expressing cells was (less) compared with that in control cells. #P<0.05 when p-Smad1/5/8 in PPM1A-expressing cells was (less) compared with that in control cells. Figure 4: DNA damage impeded SXS dephosphorylation by interfering with Smad1–PPM1A interaction. ( a ). DNA damage inhibited the dephosphorylation of nuclear Smad1/5/8. MEFs were treated with Dox for 4 h and then cultured in serum-free medium for different periods of time. The cells were collected and fractionated into cytoplasmic and nuclear fractions. Right panel: quantification of p-Smad1/5/8 that was normalized to lamin A or tubulin. The level of p-Smad1 at time 0 for untreated cells were set at 100%. All data were presented as mean±s.e.m. ( n =3) and were statistically assessed using Student's t -test. # P <0.05 when the level of p-Smad1 in Dox-treated cells was compared with that in untreated cells. ( b ) DNA damage inhibited the interaction between PPM1A and Smad1. MEFs were treated with Dox for different periods of time, collected and fractionated into the cytoplasmic and nuclear fractions, and then Smad1 was immunoprecipitated. Co-immunoprecipitated PPM1A was detected by western blot. ( c ) DNA damage inhibited the interaction between PPM1A and Smad1 in a S239 dependent manner. Flag-tagged Smad1 or Smad1S239A was expressed in 293T cells, which were treated with Dox for 6 h, and nuclear fractions were immunoprecipitated with anti-Flag conjugated beads. Same amounts of purified PPM1A proteins were added to the beads carrying Smad1 and incubated overnight. The bound PPM1A was detected by western blot. ( d ) Overexpression of PPM1A inhibited DNA damage-induced Smad1 upregulation. MEFs were infected with retrovirus expressing PPM1A, selected for 3 days, and then treated with Dox. Smad1 and p-Smad1 were detected by western blot analysis. Right panel: quantification of p-Smad1/5/8 and Smad1 that was normalized to actin. The levels of Smad1 or p-Smad1 at time 0 for vector-infected cells were set at 100%. All data were presented as mean± s.e.m. ( n =3) and were statistically assessed using Student's t -test. * P <0.05 when Smad1 in PPM1A-expressing cells was (less) compared with that in control cells. # P <0.05 when p-Smad1/5/8 in PPM1A-expressing cells was (less) compared with that in control cells. Full size image PPM1A, an interacting partner of Smad1, is one of the well-studied phosphatases responsible for SXS dephosphorylation [34] , [35] , [36] , [37] , [38] . Strikingly, Dox treatment disrupted the interaction between endogenous PPM1A and Smad1, especially for nuclear Smad1 ( Fig. 4b ). Binding assays, using bacteria-expressed PPM1A and immunoprecipitated Smad1, confirmed the inhibitory effect of Dox on Smad1–PPM1A interaction, but not S239A Smad1–PPM1A interaction ( Fig. 4c ). Moreover, overexpression of PPM1A delayed Dox-induced Smad1 SXS phosphorylation and compromised the level of SXS phosphorylation. Similar to BMPRIA deficiency, PPM1A overexpression led to a modest upregulation of Smad1 ( Figs 2a and 4d ). However, the Dox-induced Smad1 upregulation was largely inhibited by PPM1A overexpression ( Fig. 4d ). These results, together with the findings that Dox inhibited Smad1 SXS dephosphorylation and disrupted PPM1A–Smad1 interaction, suggest that PPM1A has a role in promoting Smad1 activation and upregulation in DDR. The incomplete effect of PPM1A overexpression on Smad1 activation and upregulation in DDR (compared with BMPRIA deficiency) suggest that other protein phosphatases might also be involved. Smad1 activation/upregulation is required for p53 induction Microarray analysis of gene expression profiles of Bmpr1a −/− and control ES cells at the basal level and in response to Dox treatment identified some of p53 target genes including p21 (Cdkn1a), Jun, Sfn, Myc, Pmaip1, Btg2, Ddr1, Tnfrsf10b, Traf1, IGFBP3, EGFR, MMP2, Trp53inp1, and Trp53inp2 that were suboptimally induced. This implies a link between BMP-Smad1 signalling and p53. Indeed, we found that inhibition of BMP-Smad1 signalling with noggin and chordin or BMPRIA deficiency resulted in a decrease in p53 induction in response to genotoxic stress ( Fig. 5a,b ), although BMP2 itself did not alter the levels of p53 ( Fig. 2a ), suggesting that activation of Smad1 has a necessary role in DNA damage-induced p53 induction. More importantly, Smad1 knockdown or deletion of Smad1 in Smad1f/f MEFs with retrovirus expressing Cre also led to a decrease in p53 induction by Dox, with the defect in Smad1 −/− MEFs being rescued by reconstitution with WT Smad1 or Smad1 SD mutant, but not Smad1 SA mutant ( Fig. 5c,d ), suggesting that Smad1 upregulation and S239 phosphorylation have a role in p53 expression in response to Dox. Real-time PCR analysis showed that deletion of Smad1 in Smad1f/f MEFs significantly reduced Dox-induced expression of p53 target genes p21, Mdm2, and Bax ( Fig. 5e ). However, no alteration in p53 mRNA levels was observed in the absence of Smad1 in MEFs ( Fig. 5f ). Instead, Smad1 seems to regulate p53 stability, as knockdown of Smad1 in primary MEFs led to an accelerated p53 turnover, with T 1/2 decreased from 10.3 min to 3.5 min ( Fig. 5g ). 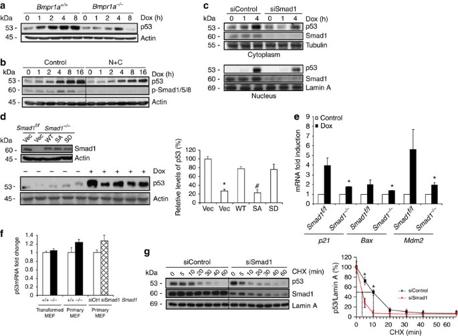Figure 5: Smad1 and S239 phosphorylation were required for optimal p53 expression. (a)Bmpr1a−/−ES cells showed reduced p53 induction in response to Dox. (b) MEFs pretreated with noggin and chordin showed reduced p53 induction in response to Dox. (c) Smad1 knockdown led to reduced p53 upregulation in response to Dox. WT MEFs transfected with control or Smad1 siRNAs were treated with Dox, and fractionated into cytoplasmic and nuclear fractions. The levels of p53 were determined by western blot analysis. (d) Smad1 WT, SD mutant, but not SA mutant Smad1, could rescue the decrease in p53 induction inSmad1−/−MEFs. Cells were treated with 1 μM Dox for 4 h. Upper left panel: expression of WT and mutant Smad1 inSmad1−/−MEFs. Bottom left: p53 induction in response to Dox in WT,Smad1−/−and reconstituted MEFs. Right panel: quantification data. All data were presented as mean±s.e.m. (n=3) and were statistically assessed using Student'st-test. *P<0.05 when p53 inSmad1−/−cells was compared with WT cells. #P<0.05 when p53 in Smad1 SA reconstituted cells was compared with WT Smad1 reconstitutedSmad1−/−cells. (e) Smad1 knockdown in MEFs impeded Dox-induced expression of p53 target genes. All data were presented as means±s.e.m. (n=3) and were statistically assessed using Student'st-test. *P<0.05 when compared with those in WT cells in the presence of Dox. (f) Real-time PCR analysis showed no significant change in the levels of p53 mRNA when Smad1 is deleted or knocked down. (g) Smad1 deletion resulted in an enhanced p53 turnover. MEFs were transfected with control or Smad1 siRNAs for 2 days. The cells were treated with cycloheximide (CHX) and the protein levels of p53 were determined by western blot analysis. Right panel: quantification data. The levels of p53 at time 0 was set at 100%. All data were presented as mean ±s.e.m. (n=3) and were statistically assessed using Student'st-test. *P<0.05 when the level of p53 in Smad1 siRNA transfected cells was compared with cells transfected with control siRNA. Figure 5: Smad1 and S239 phosphorylation were required for optimal p53 expression. ( a ) Bmpr1a −/− ES cells showed reduced p53 induction in response to Dox. ( b ) MEFs pretreated with noggin and chordin showed reduced p53 induction in response to Dox. ( c ) Smad1 knockdown led to reduced p53 upregulation in response to Dox. WT MEFs transfected with control or Smad1 siRNAs were treated with Dox, and fractionated into cytoplasmic and nuclear fractions. The levels of p53 were determined by western blot analysis. ( d ) Smad1 WT, SD mutant, but not SA mutant Smad1, could rescue the decrease in p53 induction in Smad1 −/− MEFs. Cells were treated with 1 μM Dox for 4 h. Upper left panel: expression of WT and mutant Smad1 in Smad1 −/− MEFs. Bottom left: p53 induction in response to Dox in WT, Smad1 −/− and reconstituted MEFs. Right panel: quantification data. All data were presented as mean±s.e.m. ( n =3) and were statistically assessed using Student's t -test. * P <0.05 when p53 in Smad1 −/− cells was compared with WT cells. # P <0.05 when p53 in Smad1 SA reconstituted cells was compared with WT Smad1 reconstituted Smad1 −/− cells. ( e ) Smad1 knockdown in MEFs impeded Dox-induced expression of p53 target genes. All data were presented as means±s.e.m. ( n =3) and were statistically assessed using Student's t -test. * P <0.05 when compared with those in WT cells in the presence of Dox. ( f ) Real-time PCR analysis showed no significant change in the levels of p53 mRNA when Smad1 is deleted or knocked down. ( g ) Smad1 deletion resulted in an enhanced p53 turnover. MEFs were transfected with control or Smad1 siRNAs for 2 days. The cells were treated with cycloheximide (CHX) and the protein levels of p53 were determined by western blot analysis. Right panel: quantification data. The levels of p53 at time 0 was set at 100%. All data were presented as mean ±s.e.m. ( n =3) and were statistically assessed using Student's t -test. * P <0.05 when the level of p53 in Smad1 siRNA transfected cells was compared with cells transfected with control siRNA. Full size image Smad1 interacts with p53 and inhibits p53 ubiquitination p53 stability is mainly regulated by the E3 ligase Mdm2, which ubiquitinates p53 in the nucleus and promotes its degradation [39] . Smad1 may stabilize p53 by regulating Mdm2-mediated p53 ubiquitination. We found that Smad1 did not affect the interaction between p53 and Mdm2 ( Fig. 6a ). However, co-immunoprecipitation of ectopically expressed or endogenous Smad1 and p53 showed that Smad1 did form a complex with p53 at the basal levels ( Fig. 6b,c ), and DNA damage promoted the interaction between p53 and Smad1, but not the interaction between p53 and Smad1 SA mutant ( Fig. 6d ), suggesting a role for S239 phosphorylation in enhancing Smad1–p53 interaction. More importantly, Smad1 seemed to obstruct the action of Mdm2, as Smad1 dampened Mdm2-mediated p53 ubiquitination in H1299 and HEK293 cells, while Smad1 itself was not ubiquitinated by Mdm2 ( Fig. 6e ). In vitro ubiquitination assays using purified proteins confirmed that Smad1 could inhibit Mdm2-mediated p53 ubiquitination ( Fig. 6f ). These results, together with the finding that Smad1 knockdown led to enhanced turnover of p53 ( Fig. 5g ), suggest that Smad1 binds to p53 and interferes with p53 ubiquitination and degradation. 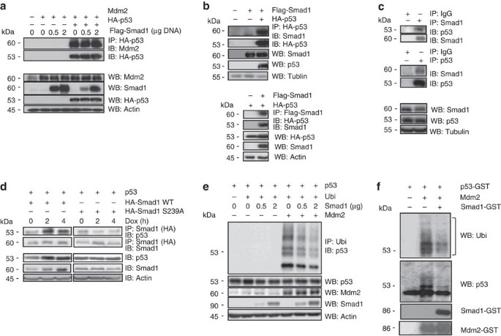Figure 6: Smad1 interacted with p53 and inhibited Mdm2-mediated p53 destabilization. (a) Ectopic expression of Smad1 did not affect the interaction between p53 and Mdm2. Smad1 with different amount of DNA, Mdm2 and p53 were transfected into 293T cells. p53 was immunoprecipitated by anti-HA antibodies and the associated Mdm2 was detected by western blot analysis. (b) Physical interaction of ectopically expressed Smad1 and p53 in 293T cells. Upper panel: p53 was immunoprecipitated with anti-HA antibodies and the associated Smad1 was detected by western blot analysis; lower panel: Smad1 was immunoprecipitated with anti-Flag antibodies and the associated p53 was detected by western blot analysis. Smad1 and p53 form a complex at the basal levels. (c) Endogenous Smad1 interacts with p53 in MEFs. Upper panel: endogenous Smad1 was immunoprecipitated with anti-Smad1 antibodies and the associated p53 was detected by western blot analysis; middle panel: endogenous p53 was immunoprecipitated with anti-p53 antibodies and the associated Smad1 was detected by western blot analysis; bottom panel: the levels of Smad1 and p53. (d) Dox treatment led to enhanced complex formation between p53 and Smad1, but not S239A Smad1. A total of 6 μg of DNA constructs were transfected into 293T cells for this assay. Because of the variation of the protein levels of transfected genes, we only did the comparison between 2/4 h to time 0 for WT or SA Smad1. (e) Smad1 repressed Mdm2-mediated p53 ubiquitination. Flag-p53, HA-ubiquitin and Mdm2, together with Smad1, were expressed in H1299 cells, which were treated with 10 μM of MG132 for 4 h before being collected. Ubiquitinated proteins were immunoprecipitated with anti-HA antibodies. Ubiquitinated p53 was detected by western blot using anti-p53 antibodies. (f)In vitroubiquitination assay showing that Smad1 was able to inhibit Mdm2-mediated p53 ubiquitination. Figure 6: Smad1 interacted with p53 and inhibited Mdm2-mediated p53 destabilization. ( a ) Ectopic expression of Smad1 did not affect the interaction between p53 and Mdm2. Smad1 with different amount of DNA, Mdm2 and p53 were transfected into 293T cells. p53 was immunoprecipitated by anti-HA antibodies and the associated Mdm2 was detected by western blot analysis. ( b ) Physical interaction of ectopically expressed Smad1 and p53 in 293T cells. Upper panel: p53 was immunoprecipitated with anti-HA antibodies and the associated Smad1 was detected by western blot analysis; lower panel: Smad1 was immunoprecipitated with anti-Flag antibodies and the associated p53 was detected by western blot analysis. Smad1 and p53 form a complex at the basal levels. ( c ) Endogenous Smad1 interacts with p53 in MEFs. Upper panel: endogenous Smad1 was immunoprecipitated with anti-Smad1 antibodies and the associated p53 was detected by western blot analysis; middle panel: endogenous p53 was immunoprecipitated with anti-p53 antibodies and the associated Smad1 was detected by western blot analysis; bottom panel: the levels of Smad1 and p53. ( d ) Dox treatment led to enhanced complex formation between p53 and Smad1, but not S239A Smad1. A total of 6 μg of DNA constructs were transfected into 293T cells for this assay. Because of the variation of the protein levels of transfected genes, we only did the comparison between 2/4 h to time 0 for WT or SA Smad1. ( e ) Smad1 repressed Mdm2-mediated p53 ubiquitination. Flag-p53, HA-ubiquitin and Mdm2, together with Smad1, were expressed in H1299 cells, which were treated with 10 μM of MG132 for 4 h before being collected. Ubiquitinated proteins were immunoprecipitated with anti-HA antibodies. Ubiquitinated p53 was detected by western blot using anti-p53 antibodies. ( f ) In vitro ubiquitination assay showing that Smad1 was able to inhibit Mdm2-mediated p53 ubiquitination. Full size image A role for Smad1 in DDR and cell transformation The above studies show that DNA damage promotes Smad1 activation and upregulation, and lack of BMP-BMPRIA or Atm not only impedes Smad1 activation but also leads to decrease of Smad1 protein levels. To test the function of Smad1 activation, which is required for Dox-induced Smad1 upregulation, in DDR, we blocked BMPs activation with noggin and chordin or BMPRIA deficiency and found that inhibition of Smad1 activation rendered the cells resistance to Dox-induced cell death ( Supplementary Fig. S5a,b ). This is consistent with reduced p53 induction in the presence of noggin and chordin or BMPRIA deficiency ( Fig. 5a,b ). We then tested the possible effects of the levels of Smad1 in DDR and found that ectopic expression of Smad1 slowed down cell proliferation whereas Smad1 deficiency resulted in opposite effects at the basal levels in MEFs ( Supplementary Fig. S6 ). Moreover, ectopic expression of Smad1 sensitized the cell death response to DNA damage ( Fig. 7a ), whereas Smad1 deficiency renders the cell resistance to Dox-induced cell death ( Fig. 7b ). This defect in Smad1 −/− MEFs could be rescued by WT Smad1 or the Smad1 SD mutant, but not the Smad1 S239A mutant ( Fig. 7b , for Smad1 protein levels, see Fig. 5d ). To determine a possible role of p53 in Smad1-regulated cell death, we increased the levels of p53, which was decreased in Smad1 −/− cells, and found this could promote cell death response to Dox ( Fig. 7b ). Moreover, overexpression of Smad1 only showed a minor effect in the cell death response to Dox in the absence of p53 ( Fig. 7b ), suggesting that p53 contributes to Smad1's function in DDR. These findings, taken together, suggest that both Smad1 activation and upregulation have an important role in DDR. 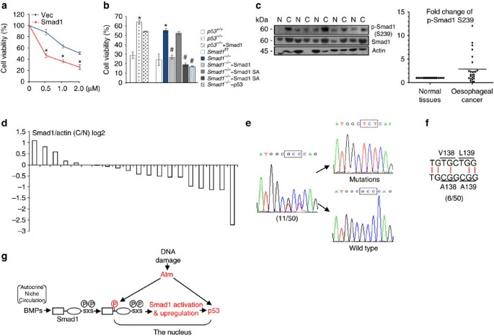Figure 7: Smad1 has a role in the DDR and tumorigenesis. (a) MEFs overexpressing Smad1 showed increased cell death rates in response to DNA damage. The MEFs were challenged with Dox and the numbers of viable cells were determined by WST-1 assay. All data were presented as mean±s.e.m. (n=3) and were statistically assessed using Student'st-test. *P<0.05 when cell survival in Smad1-ovexpressing cells was compared with the vector-infected cells. (b).Smad1−/−MEFs showed resistance to Dox-induced cell death. Reconstitution ofSmad1−/−MEFs with WT Smad1, Smad1 KD, or overexpressed p53, but not with Smad1 S239A, restored the cell death defects. All data were presented as mean±s.e.m. (n=3) and were statistically assessed using Student'st-test. *P<0.05 when cell survival in −/− cells was compared with their respective wild type. #P<0.05 when cell survival in reconstituted cells was compared withSmad1−/−cells. (c). Analysis of Smad1 S239 phosphorylation in 24 oesophageal cancer samples (C) and matched normal tissues (N). Left panel: representative western blot results of the protein and S239 phosphorylation levels of Smad1 in oesophageal cancer samples (C) compared with matched normal tissues (N). Right panel: quantification results with Actin as a loading control. The p-S239 levels of normal tissues were set at 1. (d). Quantification results of the protein levels of Smad1 in 20 gastric cancer samples. (e). Sequencing results of gastric cancer samples to show the mutations at S239 in Smad1 and the cloned DNA of the gastric cancer samples (both WT and mutant alleles). (f). Gastric cancer samples also show mutations that lead to V138A and L139A substitutions in Smad1 protein. (g). A working model showing how genotoxic stress activates Smad1 and how Smad1 promotes p53 induction to suppress tumorigenesis. BMPs activate Smad1 (SXS phosphorylation), which is translocated into the nucleus. On DNA damage, activated Atm phosphorylates SXS-phosphorylated Smad1 in the nucleus, which disrupts Smad1–PPM1A interaction and promotes Smad1–p53 interaction, leading to enhanced Smad1 activation and upregulation and p53 stabilization. Figure 7: Smad1 has a role in the DDR and tumorigenesis. ( a ) MEFs overexpressing Smad1 showed increased cell death rates in response to DNA damage. The MEFs were challenged with Dox and the numbers of viable cells were determined by WST-1 assay. All data were presented as mean±s.e.m. ( n =3) and were statistically assessed using Student's t -test. * P <0.05 when cell survival in Smad1-ovexpressing cells was compared with the vector-infected cells. ( b ). Smad1 −/− MEFs showed resistance to Dox-induced cell death. Reconstitution of Smad1 −/− MEFs with WT Smad1, Smad1 KD, or overexpressed p53, but not with Smad1 S239A, restored the cell death defects. All data were presented as mean±s.e.m. ( n =3) and were statistically assessed using Student's t -test. * P <0.05 when cell survival in −/− cells was compared with their respective wild type. # P <0.05 when cell survival in reconstituted cells was compared with Smad1 −/− cells. ( c ). Analysis of Smad1 S239 phosphorylation in 24 oesophageal cancer samples (C) and matched normal tissues (N). Left panel: representative western blot results of the protein and S239 phosphorylation levels of Smad1 in oesophageal cancer samples (C) compared with matched normal tissues (N). Right panel: quantification results with Actin as a loading control. The p-S239 levels of normal tissues were set at 1. ( d ). Quantification results of the protein levels of Smad1 in 20 gastric cancer samples. ( e ). Sequencing results of gastric cancer samples to show the mutations at S239 in Smad1 and the cloned DNA of the gastric cancer samples (both WT and mutant alleles). ( f ). Gastric cancer samples also show mutations that lead to V138A and L139A substitutions in Smad1 protein. ( g ). A working model showing how genotoxic stress activates Smad1 and how Smad1 promotes p53 induction to suppress tumorigenesis. BMPs activate Smad1 (SXS phosphorylation), which is translocated into the nucleus. On DNA damage, activated Atm phosphorylates SXS-phosphorylated Smad1 in the nucleus, which disrupts Smad1–PPM1A interaction and promotes Smad1–p53 interaction, leading to enhanced Smad1 activation and upregulation and p53 stabilization. Full size image The above studies suggest that the levels of Smad1, which can be upregulated under genotoxic stress, have an important impact on cell response to DNA damage. We tested for a role of Smad1 in cell transformation and tumorigenesis and found that elevation of Smad1 impeded transformation whereas Smad1 knockdown enhanced transformation ( Supplementary Fig. S7a ). When these cells were transplanted into nude mice, it was found that overexpression of Smad1 severely inhibited tumour formation, whereas knockdown of Smad1 accelerated tumour formation ( Supplementary Fig. S7b ). However, the inhibitory effects of Smad1 overexpression on cell transformation and tumorigenesis were much less in the absence of p53 ( Supplementary Fig. S7a,b ). These findings suggest that elevation of Smad1 inhibits cell transformation, likely through p53. Smad1 in oesophageal and gastric cancer The DDR is activated during tumour progression and DDR genes are frequently mutated in human cancers. Previous studies have shown that BMP-Smad1 signalling was downregulated in human colon cancer samples [22] . We analysed oesophageal and gastric cancer samples against their matched normal tissues and found that, unlike colon cancer samples, oesophageal tumour samples (squamous cell carcinomas) showed Smad1 upregulation and enhanced S239 phosphorylation, compared with normal matched tissues ( Fig. 7c ). This is reminiscent of previously published results showing that DNA damage is activated during tumorigenesis [5] , [6] . Based on our findings ( Fig. 7a,b ), activation of Smad1 may help to suppress tumour progression in oesophagus cancer [4] . We also analysed 20 gastric tumour samples and found that gastric cancer samples in general showed a downregulation of Smad1 and compromised activation ( Fig. 7d ), similar to the colorectal cancer samples reported [22] . We, then, sequenced the linker region of Smad1 of 50 gastric cancer samples, as this region integrates various signals to control Smad1 activation. Direct sequencing of the PCR products revealed there are mutations in this region of Smad1 in cancer samples but not in normal samples. In all cases, WT sequences were also present, suggesting heterozygosity ( Fig. 7e ). Eleven out of 50 cancer samples contain GCC to TCT mutations, which result in a S239A mutation of Smad1 protein. The mutation was confirmed by sequencing of cloned PCR products ( Fig. 7e ). In addition, 6 out of 50 cancer samples contain mutations that result in V138A and L139A substitutions in Smad1 ( Fig. 7f ). These mutations in Smad1 are likely to bestow the cells with growth advantage and are thus selected. The studies of clinical samples validate a critical role of Smad1 S239 phosphorylation in human tumorigenesis. The BMP-Smad1 cascade has emerged as a novel tumour suppression pathway, but its pathological mechanisms remain elusive [21] , [22] , [23] , [25] , [26] , [27] . This study, by establishing Smad1 as a player in cell response to DNA damage, a major driving force of oncogenesis, and linking BMP-Smad1 signalling to the prominent Atm-p53 tumour suppression pathway [4] , [40] , [41] , unveils one such mechanism. Dysfunction of BMP-Smad signalling, for example, in Juvenile Polyposis or Cowden syndrome patients, results in reduced p53 induction in DDR, conferring the cells with growth advantage and increased tumorigenic potential. BMPs are crucial regulators of embryonic development and homeostasis of various adult tissues. They are shown to regulate self-renewal and/or differentiation of a number of stem cells including neural stem cells, mesenchymal stem cells, endothelial stem cells, and skin stem cells [8] , [42] , [43] , [44] . Here we show that the presence of BMPs has an important impact on how cells respond to DNA damage. Cooperation between the BMP-Smad1 pathway and the Atm-p53 pathway is necessary for the cell to elicit an optimal DDR. Previous studies by us and others have shown that nutrition and growth factors can affect the induction of p53 under genotoxic stress via the mTOR-S6 K pathway [45] , [46] , [47] . These findings, taken together, suggest that the environment of cells have a critical role in DDR and as a consequence in cell transformation and tumorigenesis. BMP-Smad signalling is tightly controlled by various negative regulators [13] , [14] , [18] . BMPs-induced activation of Smad1/5/8 is relatively transient, with Smad1 being quickly cycled back to the cytoplasm, leading to a decrease in the levels of nuclear Smad1 ( Figs 1d and 2c ) [19] , [48] . However, DNA damage leads to sustained Smad1 activation and upregulation, especially in the nucleus. Our observations, namely Dox treatment or Atm deficiency does not affect the expression of the major BMP ligands and receptors; Dox treatment does not affect the kinase activity of BMPRIA towards Smad1; and Atm does not phosphorylate BMPRIA or BMPRII, suggest that DNA damage and Atm control Smad1 activation and upregulation not via BMP ligands or receptors. Instead, our results suggest that DNA damage acts on SXS-phosphorylated Smad1 and inhibits SXS dephosphorylation, thus extending Smad1 activation and leading to Smad1 upregulation in the nucleus. The observation that BMPRIA deficiency, Smad1 SXS deletion, noggin and chordin treatment all diminished Smad1 S239 phosphorylation suggests that Dox-induced Smad1 upregulation requires sequential phosphorylation events, BMPRI-mediated SXS phosphorylation and Atm-mediated S239 phosphorylation, and a cooperation between BMP-BMPR-mediated Smad1 activation and DNA damage-activated Atm ( Fig. 7g ). These findings reveal another mechanism that activates Smad1 and further support the importance of the linker region of Smad proteins. Surprisingly, unlike BMPs, DNA damage seems not to activate the feedback regulatory mechanism by I-Smads as Dox does not activate the expression of Smad6 and Smad7, and transient knockdown of Smad6 or Smad7 does not significantly affect Dox-induced p53 expression or cell death (Liu H and Li B, unpublished results). It has been previously reported that p53 interacts with Smad2/3 to regulate the expression of genes that control TGFβ-mediated mesoderm induction as well as its cytostatic effects in mammalian cells [49] , and this interaction could be enhanced by RTK-Ras-CK1ɛ/δ- mediated S9 phosphorylation of p53 [50] , [51] , [52] 50–52). In addition, DNA damage has been reported to activate TGFβ-Smad2/3 signalling and that TGFβ and Smad7 have a role in activation of Atm, yet, Atm-p53 activation was shown to be independent of Smad2/3 (refs 53 , 54 , 55 , 56 , 57 ). However, our study revealed that Smad1 is preferentially activated in response to Dox in primary cells and several cell lines and that Smad1–p53 interaction has a role in the DDR in mammalian cells. S239 phosphorylation and Smad1 upregulation promote Smad1–p53 complex formation and facilitate p53 stabilization in the nucleus, which, in turn, constrains cell propagation. In addition, complex formation between these two proteins might affect the activity of each transcription factor, which awaits further investigation. Taken together, ours and others' work suggest that both TGFβ and BMPs have a role in the DDR. In summary, this study identified Smad1 as an additional player in the DDR, whose activation requires sequential BMPRIA-mediated SXS phosphorylation and Atm-mediated S239 phosphorylation, and leads to maximal p53 induction. The link to the prominent Atm-p53 tumour suppression pathway provides an explanation why dysfunction of BMP-Smad1 signalling results in tumorigenesis. As part of the DDR, Smad1 is found to be phosphorylated on S239 during oesophageal tumour progression and is frequently mutated in gastric cancer samples, and is activated in various tumour cell lines in response to radio- or chemo-therapy drugs. As such, Smad1 might hold promise for anti-cancer drug development. Mice and cell cultures Atm −/− , p53 −/− , Smad1 −/− MEFs were prepared as previously described [30] . Atm −/− , p53 −/− , and Balb/c nude mice were bred and used, following the guidelines of the Institute of Molecular and Cell Biology, with protocols approved by Animal Care and Use Committee, Singapore. Some Smad1 −/− MEFs was transformed with Ras V12 /E1A expressing retrovirus. MEFs, 293T, HCT116 and H1299 cells were cultured in DMEM supplemented with 10% FBS and penicillin/streptomycin in humidified atmosphere of 5% CO 2 at 37 °C. Mouse Bmpr1a −/− and normal ES cells were cultured in the presence of LIF and ES cell-certified serum. DNA damage was generated by treatment cells with 0.2–2.5 μM Dox (Calbiochem), different doses of gamma-radiation, or 5 mM hydroxyurea (Sigma), unless otherwise indicated. Transfection and retrovirus infection To transiently express a given protein, cells were transfected with lipofectamine (Life Technologies, Gaithersburg, MD, USA). For 6 cm plates, a total of 6 μg of DNA was used for transfection, whereas12 μg of DNA was used to get saturated effects. To transiently knockdown Smad1, ON-TARGETplus SMART pool siRNA were used (DHARMACON). To stably express Smad1 or PPM1A, a retroviral vector pMSCV was used. The retrovirus was produced by Plat E packaging cells. MEFs were infected with these viruses or control virus, and then selected against puromycin for 3 days, before splitted for further assays. For long-term knockdown experiment, the retrovirus carrying the short hairpin RNA against Smad1 was introduced to MEFs and selected with puromycin. Cell viability analysis To measure cell death rates, cells were plated in 96 well plates at 1×10 4 per well, and then treated with different doses of Dox for 24–48 h. Cell proliferation reagent WST-1 (Roche) was added to each well and the cells were further incubated for another 3 h at 37 °C. The absorbance was measured against a background control by microplate (ELISA) reader at 430 nm. Analysis of protein expression and localization Cells were lysed in RIPA buffer or co-immunoprecipitation buffer (20 mM Tris pH7.5, 100 mM NaCl, 0.5% NP-40, 0.5 mM EDTA) for co-immunoprecipitation experiments. Phosphatase inhibitors and protease inhibitors were added to the buffers before use. Protein concentration was determined by the Bio-Rad assay. Immunoprecipitation and immunobloting were carried out using the following antibodies: antibodies against p53 (2524,1:1000), p-p53 (Ser15) (9284, 1:1000), Lamin A/C (2032, 1:1000), p-Smad1/5/8 (9511, 1:1000), Smad1 (9743, 1:1000), Smad5 (9517, 1:500), p-Smad2 (3101, 1:1000), Smad2/3 (3102, 1:1000), p-(S/T)Q (2851, 1:500) and Tubulin (2148, 1:2000). These were purchased from Cell Signaling. Antibodies against Id1 (sc-374287, 1:500), HA (sc-161069, 1:1000), Smad8 (sc-11393, 1:500), Actin (sc-130656, 1:1000) and GST (sc-138, 1:500) were from Santa Cruz. Antibodies against Flag (F2555, 1:2000) were from Sigma. Antibodies against p-Atm (ab2888, 1:1000), BMPRIA (ab-38560, 1:1000), and PPM1A (ab94627, 1:1000) were from Abcam. Antibodies against p21 (OP76, 1:1000) and Mdm2 (OP46, 1:1000) were from Calbiochem. For confocal microscopy, cells stably expressing Smad1 or Flag-tagged Smad1 or transiently expressing Smad1 were grown overnight on glass cover-slips, subjected to Dox or BMP2 treatment, and fixed with 4% paraformaldehyde and permeabilized with 0.1% Triton X-100 for 20 min, blocked with 5% BSA for 30 min, and then incubated with anti-Flag or Smad1antibodies and FITC-conjugated secondary antibodies. Antibody production Rabbit polyclonal antibody against p-Smad1 (Ser 239) with peptide sequence CDPMTQDG[pS]QPMDTN was customer made by Open Biosystems and purified by affinity purification. In vitro kinase assay for Atm The in vitro kinase assay was performed with immunoprecipitated Atm and bacteria-expressed GST-Smad1 as the substrate, following a protocol previously described [33] . A portion of the reaction was used to determine the levels of Smad1-GST and Atm. Real-time PCR and microarray analysis Total RNA was extracted from cells with TRIzol reagent (Invitrogen) according to the manufacturer's protocol. Complementary DNAs were synthesized with 0.5 μg of total RNA using iScript cDNA Synthesis Kit (Bio-Rad). The detection and quantification of target mRNA were performed with real-time PCR. For microarray analysis, probe labelling reaction and microarray hybridization, image process, and data normalization were carried out following the manufacturer's instructions (Illumina). The log 2 ratios of each time point were then normalized for each gene to that of untreated cells (time 0) to obtain the relative expression pattern. The genes that showed substantial change after drug treatment were selected based on a twofold change of expression value across all experimental conditions. The genes out of 24,000 that met the criteria were further analysed. In vitro p53 ubiquitination assay In vitro p53 ubiquitination assay was carried out as previously described [58] . Briefly, for each reaction, 40 ng of p53-gst (Signalchem) was mixed with the following components: 100 ng E1 (UBE1-gst, Boston Biochem), 400 ng E2 (UbcH5c-gst, Boston Biochem), 2 μg Ubiquitin (Signalchem) and 500 ng Mdm2-gst (GenWay Biotech) in the presence or absence of 100 ng Smad1-gst (Signalchem). These components were incubated at 37 °C for 60 min in ubiquitination buffer (40 mM Tris, 5 mM MgCl 2 , 2 mM ATP, 2 mM DTT, pH 7.6), and the final volume was 50 μl. SDS sample buffer was added to stop the reaction and the ubiquitinated p53 was subsequently detected by western blot with antibodies against p53 (1C12, 1:1000, Cell Signaling) or ubiquitin (P4D1, 1:500, Santa Cruz). Cell transformation and tumorigenesis Primary WT or p53 −/− MEFs that stably expressed short hairpin RNA to silence Smad1, or stably overexpressed Smad1 were transformed by infection of retrovirus that expressed both E1A and Ras V12 . Two days after infection, the cells were either cultured in 5% serum DMEM for colony formation assay in which colonies were fixed by methanol and stained by Giemsa, or applied for xenografts by injecting subcutaneously (3×10 6 cells) to nude mice (BALB/c nude, 6–7-week-old). The length ( l ) and width ( w ) of the tumour were measured by a digital caliper and the tumour volumes were calculated by l × w 2 (mm 3 ). Gastric cancer sample collection and sequencing of Smad1 cDNA Gastric cancer samples and adjacent normal tissues were obtained at the time of surgical resection and were frozen in liquid nitrogen and stored at −80 °C until use. This study was approved by the Institutional Review Board of the Bio-X Institutes, Shanghai Jiao Tong University Shanghai, China. Frozen tissues were used for both DNA and RNA extraction with standard protocols. RNA samples were reverse transcribed using Qiagen RT–PCR kit. The Smad1 cDNA (the linker region) was amplified using 5′-TGTCATTTACTGCCGTGTGTGG-3′ and 5 ′ -GCAGCCCAAGGCAGAAACGGT-3 ′, which was directly sequenced with primers 5 ′ -CGATCTTCAGAGCCACCATG-3 ′ and 5 ′ -GTTGGAAGGATCAGTGAAACC-3 ′. For tumour samples that contain Smad1 mutations, the PCR products were subcloned into pBluescript II SK and then sequenced using T3 and T7 primers. Image quantification and statistical analysis All the presented experiments have been repeated at least three times, with similar results obtained. The representative results were presented. For quantification, western blot results were scanned with a Molecular Dynamics scanning densitometer. The relative levels of proteins of interest were then determined by measuring the intensity of the corresponding bands, which were normalized to the internal controls. Statistical analysis was performed using Student's t -test. Significant association was defined when P <0.05 compared with control. Accession codes: The microarray data have been deposited in the GEO database under the accession code GSE36843 . How to cite this article: Chau, J.F.L. et al . A crucial role for bone morphogenetic protein-Smad1 signalling in the DNA damage response. Nat. Commun. 3:836 doi: 10.1038/ncomms1832 (2012).